A Munc13-like protein inArabidopsismediates H+-ATPase translocation that is essential for stomatal responses Plants control CO 2 uptake and water loss by modulating the aperture of stomata located in the epidermis. Stomatal opening is initiated by the activation of H + -ATPases in the guard-cell plasma membrane. In contrast to regulation of H + -ATPase activity, little is known about the translocation of the guard cell H + -ATPase to the plasma membrane. Here we describe the isolation of an Arabidopsis gene, PATROL1 , that controls the translocation of a major H + -ATPase, AHA1, to the plasma membrane. PATROL1 encodes a protein with a MUN domain, known to mediate synaptic priming in neuronal exocytosis in animals. Environmental stimuli change the localization of plasma membrane-associated PATROL1 to an intracellular compartment. Plasma membrane localization of AHA1 and stomatal opening require the association of PATROL1 with AHA1. Increased stomatal opening responses in plants overexpressing PATROL1 enhance the CO 2 assimilation rate, promoting plant growth. Stomatal pores, formed by pairs of guard cells, serve as major gateways for gas exchange between plants and their environments [1] . Opening of stomata is stimulated by low CO 2 concentrations and light, whereas stomatal closure occurs in response to high CO 2 , darkness and shortage of water. Guard cells integrate these signals and appropriately adjust the stomatal pore apertures to optimize growth performance [2] , [3] . Stomatal opening is driven by an increase in guard-cell turgor when plasma membrane H + -ATPases are activated through phosphorylation and induce membrane hyperpolarization facilitating K + entry into the guard cells [4] , [5] . Although the activity of plasma membrane H + -ATPases is modulated by various physiological signals, there is little evidence that these factors alter the abundance of H + -ATPase in the plasma membrane [6] . Here we describe a Munc13 ortholog named PATROL1 that in Arabidopsis controls the tethering of an H + -ATPase, AHA1 [7] , to the plasma membrane, and demonstrate that PATROL1 function is essential for stomatal opening in response to low [CO 2 ] and light. The patrol1 mutation impairs the stomatal opening response Leaf temperature acts as a convenient indicator of transpiration and can help detect mutants with altered stomatal control [8] , [9] . Arabidopsis ht mutants were identified by higher leaf temperature than the wild type (WT) under low CO 2 conditions, as visualized by infrared imaging [9] ( Fig. 1a ). One of them, a recessive mutant originally referred to as ht2 and here renamed patrol1 ( proton ATPase translocation control 1) , was impaired in CO 2 -dependent leaf temperature change ( Fig. 1a ) as well as in stomatal opening in response to low [CO 2 ] ( Fig. 1b ). The stomatal density of 3-week-old leaves was similar in WT and patrol1 plants (136±23.4 and 132±23.6 stomata per mm 2 in WT and patrol1 , respectively; means±s.d. ; n =20 leaves). Thus, the high leaf temperature at low [CO 2 ] in patrol1 could not be explained by stomatal density, but by a reduction of stomatal aperture. 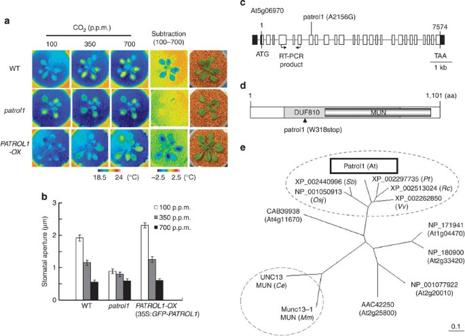Figure 1: TheArabidopsisMunc13-like protein PATROL1 is required for stomatal CO2response. (a) Three-week-old plants were subjected to the indicated [CO2]. The subtractive images show changes in leaf temperature in response to the transfer from high to low [CO2]. (b) CO2response of stomatal aperture in WT,patrol1mutants and 35S:GFP–PATROL1. Three-week-old plants were incubated at the indicated [CO2]. Data are means±s.e.m. (n=60) of three independent experiments. (c) Structure of thePATROL1gene.PATROL1consists of 27 exons (white boxes); black boxes highlight the 5′ and 3′ untranslated regions, respectively. Arrows indicate regions used in RT-PCR (Supplementary Figs S2, S4). (d)PATROL1encodes a protein of unknown function with a MUN domain. DUF810 (IPR008528; 194–865 aa), MUN (428–1042 aa). (e) Phylogenetic relationships based on amino-acid sequence similarities between MUN domain-containing proteins and the MUN domains of Unc13/Munc13 proteins (UNC13-MUN (Ce:C. elegans), Munc13-1 MUN (Mm:Mus musculus)), as determined with CLUSTAL X. At,Arabidopsis thaliana; Rc,Ricinus communis; Vv,Vitis vinifera; Osj,Oryza sativa subsp.japonica; Sb,Sorghum bicolor; Pt,Populus trichocarpa. Figure 1: The Arabidopsis Munc13-like protein PATROL1 is required for stomatal CO 2 response. ( a ) Three-week-old plants were subjected to the indicated [CO 2 ]. The subtractive images show changes in leaf temperature in response to the transfer from high to low [CO 2 ]. ( b ) CO 2 response of stomatal aperture in WT, patrol1 mutants and 35S: GFP–PATROL1 . Three-week-old plants were incubated at the indicated [CO 2 ]. Data are means±s.e.m. ( n =60) of three independent experiments. ( c ) Structure of the PATROL1 gene. PATROL1 consists of 27 exons (white boxes); black boxes highlight the 5′ and 3′ untranslated regions, respectively. Arrows indicate regions used in RT-PCR ( Supplementary Figs S2, S4 ). ( d ) PATROL1 encodes a protein of unknown function with a MUN domain. DUF810 (IPR008528; 194–865 aa), MUN (428–1042 aa). ( e ) Phylogenetic relationships based on amino-acid sequence similarities between MUN domain-containing proteins and the MUN domains of Unc13/Munc13 proteins (UNC13-MUN (Ce: C. elegans ), Munc13-1 MUN (Mm: Mus musculus )), as determined with CLUSTAL X. At, Arabidopsis thaliana ; Rc, Ricinus communis ; Vv, Vitis vinifera ; Osj, Oryza sativa subsp.japonica ; Sb, Sorghum bicolor ; Pt, Populus trichocarpa . Full size image PATROL1 encodes a protein with MUN domain The PATROL1 locus was mapped to a location between the Cereon single-nucleotide polymorphism marker, CER438918, and the original molecular marker moj9-47976, on chromosome 5 ( Supplementary Fig. S1 ). Sequencing of this 47-kb region revealed that At5g06970 harboured a point mutation at nucleotide 2,156 that resulted in the exchange of Trp-318 for a stop codon ( Fig. 1c,d ). The 3.8-kb PATROL1 cDNA fragment expressed under the control of the CaMV 35S promoter complemented the smaller mutant phenotype and restored the CO 2 response in stably transformed patrol1 (35S: PATROL1 ) ( Supplementary Fig. S2 ). This indicates that PATROL1 is At5g06970, which encodes an uncharacterized protein with a Domain of Unknown Function 810 (DUF810) ( Fig. 1c ; InterPro; http://www.ebi.ac.uk/interpro/ ) of 1,101 amino acids. Plant proteins that have a MUN domain have been classified as DUF810 ( Fig. 1d ). Munc13 proteins are crucial components in neurotransmitter release in animals, controlling the priming of synaptic vesicles to the release-ready state [10] , [11] . Intracellular membrane fusion is generally dependent on the activities of SNARE complexes [12] . A large α-helical domain of mammalian Munc13-1, the MUN domain, dramatically accelerates the transition from the closed Syntaxin-1/Munc18-1 complex to the SNARE complex [13] , and is sufficient for the activity of Munc13-1 in synaptic vesicle priming [14] . MUN domains are found in diverse proteins from animals, plants and fungi [15] , [16] . Munc13 proteins in animals have extensive conserved sequences and domains in addition to the MUN domain [16] . We compared the amino-acid sequences of the MUN domains of two representative Munc13 proteins. The animal MUN domains exhibit weak amino-acid identities with PATROL1 ( Fig. 1e ; 16% in Unc13-MUN ( C. elegans ) and 8% in Munc13-MUN ( Mus musculus )). The sequence identities of PATROL1 with five other Arabidopsis DUF810 members are not high (17–32%; Fig. 1e , Supplementary Fig. S3 ). On the other hand, higher plants including monocots and dicots have PATROL1 orthologues with highly conserved homologies distributed across the entire sequences (identities; 66–76%; Fig. 1e , Supplementary Fig. S3 ), suggesting an essential function. Computational biology and available three-dimensional (3D) structures indicate structural similarity between MUN domains of Munc13-related proteins including PATROL1 and other distantly related vesicle tethering factors such as the Exocyst, GARP, COG and Dsl1p complexes [16] , [17] . This suggests that PATROL1 may have a conserved function in intracellular membrane fusion. Expression pattern of PATROL1 in Arabidopsis To examine the expression patterns of PATROL1 , we used the PATROL1 promoter to drive expression of the GUS reporter (p PATROL1 :: GUS ; Supplementary Fig. S4a–f ), and RT-PCR analysis with gene-specific primers ( Fig. 1c , Supplementary Fig. S4g,h ). PATROL1 was expressed in the whole plant, including guard cells ( Supplementary Fig. S4 ). Global gene expression analysis of microarrays indicated that other DUF810 member genes in Arabidopsis were expressed mainly in floral organs ( At1g04470 and At2g33420 ) or in the whole plant ( At2g20010 , At2g25800 and At4g11670 ), similar to PATROL1 [18] . Two closely related genes ( At2g33420 and At4g11670 ) were expressed especially in mature pollen and pollen tubes, suggesting roles in pollen germination and tube growth [19] . Compared to other DUF810 member genes with pleiotropic expression, PATROL1 expression levels appeared relatively high [18] , and the loss-of-function mutation in PATROL1 impaired stomatal movement ( Fig. 1b ) and caused growth retardation ( Supplementary Fig. S2 ), raising the possibility that PATROL1 has a major function in stomatal response and plant growth. Environmental conditions alter PATROL1 subcellular distribution We generated transgenic plants expressing green fluorescent protein (GFP) fused to the N terminus of the full-length PATROL1 protein (GFP–PATROL1) to determine the intracellular localization of PATROL1. The GFP–PATROL1 rescued the patrol1 mutant phenotype; the plants showed increased sensitivity to low [CO 2 ] due to overexpression of the transgenes ( Fig. 1a,b , Supplementary Fig. S2 ). The lipophilic dye FM4-64 is internalized in living cells through endocytosis and can be used to visualize the endocytic pathway from the plasma membrane to the tonoplast [20] , [21] . Two minutes after the transfer of GFP–PATROL1 transgenic plants into FM4-64 buffer, the fluorescent dye exhibited a punctate pattern typical of endosomes with little or no vacuolar staining in hypocotyl epidermal cells ( Fig. 2a,b ). The FM4-64 signal partially colocalized with the GFP–PATROL1 fluorescence signal ( Fig. 2b ), indicating that GFP–PATROL1 resides in an endosomal compartment. This finding paralleled results from mouse brain cells, where signals from Munc13-1-EYFP and FM4-64 also colocalized [22] . When incubated in the dark for 72 h, numerous small structures showing GFP–PATROL1 fluorescence were observed in the guard cells of leaves in transgenic plants ( Fig. 2c,d ; dark); their number decreased after 30 min in the light ( Fig. 2c,d ; light for 30 min). The structures were rare in the guard cells of well-watered and irradiated plants, when most of the GFP–PATROL1 fluorescence was detected in close proximity to the plasma membrane ( Fig. 2e,f ; detached for 0 min). Within 30 min after detachment of the leaves, small fluorescent structures were observed inside the cell ( Fig. 2e,f ; detached for 30 min). These findings suggest that GFP–PATROL1 moved reversibly between the cytoplasm and the plasma membrane depending on environmental conditions. 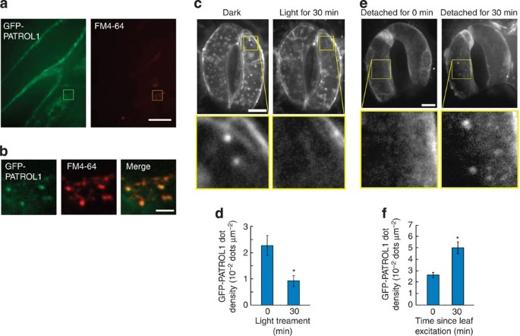Figure 2: Endosome-localized PATROL1 changes its distribution in response to environmental conditions. (a,b) Endosomal localization of GFP–PATROL1. Images of GFP–PATROL1 (green) and FM4-64 (red) in hypocotyl epidermal cells. The yellow square in (a) shows the part of the image that is enlarged in (b). Scale bars indicate 20 μm in (a) and 2 μm in (b). (c,d) GFP–PATROL1 localization changes in response to irradiation. Data are means±s.e.m. of four to seven independent guard cells. (e,f) GFP–PATROL1 localization changes in response to drought stress after leaf detachment. Data are means±s.e.m. of three independent guard cells. Asterisks indicate statistical significance (*P<0.05) as determined by Welch’st-test. Scale bars=5 μm in (c) and (e). Figure 2: Endosome-localized PATROL1 changes its distribution in response to environmental conditions. ( a , b ) Endosomal localization of GFP–PATROL1. Images of GFP–PATROL1 (green) and FM4-64 (red) in hypocotyl epidermal cells. The yellow square in ( a ) shows the part of the image that is enlarged in ( b ). Scale bars indicate 20 μm in ( a ) and 2 μm in ( b) . ( c , d ) GFP–PATROL1 localization changes in response to irradiation. Data are means±s.e.m. of four to seven independent guard cells. ( e , f ) GFP–PATROL1 localization changes in response to drought stress after leaf detachment. Data are means±s.e.m. of three independent guard cells. Asterisks indicate statistical significance (* P <0.05) as determined by Welch’s t -test. Scale bars=5 μm in ( c ) and ( e ). Full size image Mutation of PATROL1 causes altered localization of AHA1 If PATROL1 has a role in intracellular membrane traffic, it might control the localization of ion transporters that are crucial to stomatal opening (for example, plasma membrane H + -ATPases). Stomatal opening is initiated by hyperpolarization of the guard-cell plasma membrane caused by H + -ATPase-dependent proton efflux [5] . Membrane hyperpolarization activates inward-rectifying potassium channels and induces solute influx followed by water uptake into guard cells [4] . Arabidopsis H + -ATPase 1 (AHA1) is highly expressed in guard cells and its activation induces stomatal opening [7] , [23] . We generated transgenic plants containing a GFP–AHA1 fusion gene in the WT (AHA1/WT) and patrol1 (AHA1/ patrol1 ) background. In WT guard cells, GFP–AHA1 was localized mainly at the plasma membrane ( Fig. 3a ) as expected [24] . The internalization rate calculated from the number of guard cells that exhibited small fluorescent structures in their cytosol was 80% in AHA1/ patrol1 transgenic plants ( Fig. 3a,b ). This rate was significantly higher than that of AHA1/WT transgenic plants (8%; Fig. 3a,b ), indicating that PATROL1 affects AHA1 localization to the plasma membrane. The slow anion channel SLAC1 contributes to anion efflux from guard cells and causes membrane depolarization, resulting in stomatal closure [25] , [26] . We compared the distribution of SLAC1–GFP fluorescence in transgenic WT and patrol1 plants. Little internalization was observed in the guard cells of SLAC1–GFP transgenic plants even in the patrol1 background (SLAC1/WT, 1%; SLAC1/ patrol1 , 3%; Fig. 3a,b ). We examined another transporter, aquaporin PIP1a, which is localized in the plasma membrane of guard cells [27] . GFP–PIP2a has been used as a plasma membrane protein marker [28] , and we also detected GFP fluorescence in the plasma membrane (GFP–PIP2a/WT, Fig. 3a,b ). In the patrol1 background, the internalization rate of GFP–PIP2a was slightly increased but remained low (PIP2a/WT, 0%; PIP2a/ patrol1 , 8.6%; Fig. 3a,b ). These results indicated that PATROL1 is target-selective, as it is required for the direction of AHA1 to the plasma membrane, but less so for SLAC1 or PIP2a. We also examined the localization of the inward-rectifying potassium channel, KAT1, in patrol1 mutants. This voltage-gated channel is activated by hyperpolarization, and mediates the influx of potassium into guard cells [29] . We could only slightly detect punctate structures of KAT1–GFP fluorescence in patrol1 mutants, indicating that PATROL1 does not affect KAT1 localization to the plasma membrane (KAT1/WT, 0.6%; KAT1/ patrol1 , 1.1%; Supplementary Fig. S5 ). To our knowledge, the KAT1–GFPfluorescence in WT chloroplast envelopes that we detected has never been discussed before, but some figures in a previous report [30] showed similar localization. Among the four GFP-tagged plasma membrane-localized proteins in our transgenic plants, the fluorescence intensity of GFP–AHA1 was the strongest. As overexpressed membrane-targeted GFP fusion proteins have a propensity to form organelle aggregates as a consequence of oligomerization [31] , we examined whether the increased internalization rate of the GFP–AHA1 in the patrol1 mutant was caused by GFP. The monomeric red fluorescent protein (mRFP) contains 33 mutations compared to DsRed and was designed as a non-oligomerizing, true monomer [32] . The RFP-tagged AHA1 in the patrol1 mutant appeared as numerous punctate structures in the cytosol ( Fig. 3c ), while it exhibited an extremely low fluorescence intensity in the plasma membrane ( Fig. 3d,e ), indicating apparent mislocalization of AHA1. We further attempted to identify plasma membrane H + -ATPases in the epidermis of rosette leaves using anti-H + -ATPase antibodies (anti-AHA) ( Supplementary Fig. S6 ). The mean value of the fluorescent intensity from immunohistochemical staining in patrol1 was slightly but not statistically significantly lower than in the WT (266.1 in arbitrary unit in WT, 288.3 in arbitrary unit in patrol1 , respectively; P =0.24, Supplementary Fig. S6 ). One reason why no clear difference could be observed is that this method has the potential to detect not only plasma membrane AHA but also AHA in endosomes. Actually, intracellular localization of the H + -ATPase has been found by this method, probably due to an artifact caused by the fixation for immunohistochemical detection [33] . It also seemed extremely difficult to distinguish endosomal AHA from plasma membrane AHA in guard cell protoplast proteins and to quantify their amounts. In order to estimate the amount of functional H + -ATPases in the plasma membrane of guard cells, we investigated stomatal apertures when H + -ATPases were compulsorily activated. The fungal phytotoxin fusicoccin (FC) induces irreversible stomatal opening by the continuous activation of the plasma membrane H + -ATPases due to inhibition of their dephosphorylation in guard cells [5] , [34] . Though Arabidopsis has at least 11 plasma membrane H + -ATPases and all of which are expressed in guard cells [23] , the stomatal response to FC was severely impaired in patrol1 ( Fig. 3f ;<0.5, unpaired two-tailed t -test), suggesting that the recruitment of functional H + -ATPases to the plasma membrane was disturbed by the mutation. Thus, PATROL1 may have a crucial role in the recruitments of not only AHA1 but also of the other H + -ATPases. 35S: PATROL1 and 35S: GFP–PATROL1 transgenic plants showed rather strong FC responses indicating increased AHA level in the plasma membrane ( Fig. 3f ). To obtain further insights into the relationship between PATROL1 and AHA1, we generated transgenic plants co-expressing GFP–PATROL1 and RFP–AHA1. In hypotonic conditions, which lead to stomatal opening, RFP–AHA1 was located in the plasma membrane, while GFP–PATROL1 seemed to line the membrane ( Fig. 4a ). In hypertonic conditions, which induce stomatal closure, RFP–AHA1 partially remained in the plasma membrane and GFP–PATROL1 seemed to support it. They resided on the plasma membrane–cell wall connection spots, that is, the tips of Hechtian strands in a plasmolyzed guard cells ( Fig. 4b , arrows). These relationships suggest that PATROL1 contributes to H + -ATPase localization to the plasma membrane. 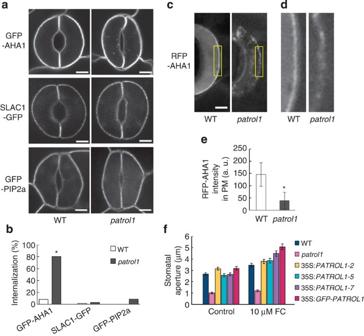Figure 3:patrol1mutation perturbs the plasma membrane localization of AHA1. (a) Optical sections showing the GFP–AHA1, SLAC1–GFP and GFP–PIP2a signals in guard cells in transgenic WT andpatrol1plants. Thepatrol1mutation caused mislocalization of GFP–AHA1, which showed as internalized dots. Scale bars=5 μm. (b) Percentages of guard cells of GFP–AHA1, SLAC1–GFP and GFP–PIP2a plants with 0.05 dots per μm2or denser. Around 197–269 guard cells were examined. Maximum intensity projection images reconstructed from serial optical sections, captured from the guard cell surface to the mid-plane with 1-μm intervals, were evalated. Asterisk indicates statistical significance (P<0.001, Ryan’s test.) (c) Optical sections of RFP–AHA1-expressing guard cells in transgenic WT andpatrol1plants. Scale bar=5 μm. (d) Enlarged sectors of images on the (c). (e) Intensities of RFP–AHA1 fluorescence in the plasma membrane. Resions of the plasma membrane were determined with cytosolic fluorescein diacetate staining. Data are mean values±s.d. of 10 independent guard cells. Asterisk indicates statistical significance (*P<0.0001, unpaired two-tailedt-test) (f) Effect of FC on stomatal opening. Data are means±s.e.m. of 60 apertures measured in three independent experiments. Figure 3: patrol1 mutation perturbs the plasma membrane localization of AHA1. ( a ) Optical sections showing the GFP–AHA1, SLAC1–GFP and GFP–PIP2a signals in guard cells in transgenic WT and patrol1 plants. The patrol1 mutation caused mislocalization of GFP–AHA1, which showed as internalized dots. Scale bars=5 μm. ( b ) Percentages of guard cells of GFP–AHA1, SLAC1–GFP and GFP–PIP2a plants with 0.05 dots per μm 2 or denser. Around 197–269 guard cells were examined. Maximum intensity projection images reconstructed from serial optical sections, captured from the guard cell surface to the mid-plane with 1-μm intervals, were evalated. Asterisk indicates statistical significance ( P <0.001, Ryan’s test.) ( c ) Optical sections of RFP–AHA1-expressing guard cells in transgenic WT and patrol1 plants. Scale bar=5 μm. ( d ) Enlarged sectors of images on the ( c ). ( e ) Intensities of RFP–AHA1 fluorescence in the plasma membrane. Resions of the plasma membrane were determined with cytosolic fluorescein diacetate staining. Data are mean values±s.d. of 10 independent guard cells. Asterisk indicates statistical significance (* P <0.0001, unpaired two-tailed t -test) ( f ) Effect of FC on stomatal opening. Data are means±s.e.m. of 60 apertures measured in three independent experiments. 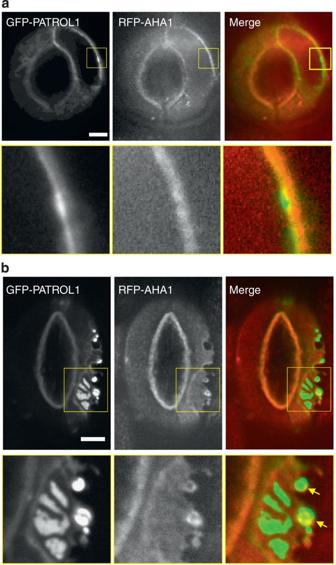Figure 4: PATROL1 lines with plasma membrane-localized AHA1. Subcellular localizations of GFP–PATROL1 and RFP–AHA1 in co-expressing transgenic plants under hypo-osmotic (a; 120 mOsM) and hyper-osmotic (b; 530 mOsM) conditions. (a,b) Enlarged images of the region enclosed in the yellow square are shown directly below. Scale bars=5 μm. (a) RFP–AHA1 in the plasma membrane was lined by PATROL1 under hypotonic condition. (b) RFP–AHA1 and GFP–PATROL1 remain at the tips of Hechtian strands in plasmolyzed guard cells. The remaining positions are indicated by arrows. Full size image Figure 4: PATROL1 lines with plasma membrane-localized AHA1. Subcellular localizations of GFP–PATROL1 and RFP–AHA1 in co-expressing transgenic plants under hypo-osmotic ( a ; 120 mOsM) and hyper-osmotic ( b ; 530 mOsM) conditions. ( a , b ) Enlarged images of the region enclosed in the yellow square are shown directly below. Scale bars=5 μm. ( a ) RFP–AHA1 in the plasma membrane was lined by PATROL1 under hypotonic condition. ( b ) RFP–AHA1 and GFP–PATROL1 remain at the tips of Hechtian strands in plasmolyzed guard cells. The remaining positions are indicated by arrows. Full size image Stomatal opening and CO 2 uptake in PATROL1-OX plants To characterize the function of PATROL1 , we compared the phenotypes of the patrol1 mutant and the PATROL1 -overexpressing line ( Supplementary Fig. S2c ). 35S: GFP–PATROL1 (hereafter PATROL1-OX ) exhibited functional complementation of patrol1, including restored sensitivity to FC ( Fig. 3f ) and low [CO 2 ] ( Fig. 1a , Supplementary Fig. S2b ) . PATROL1-OX exhibited lower leaf temperature under low [CO 2 ] than the WT due to enhanced stomatal opening ( Fig. 1a,b ). The rises in stomatal conductance in response to low [CO 2 ] and light were more rapid and reached higher maximum values (sometimes followed by oscillations) in PATROL1-OX than in the WT, whereas those in patrol1 were slow and ceased at low values ( Fig. 5a,c ). Enhanced stomatal opening responses in PATROL1-OX plants may contribute to higher CO 2 assimilation rates even under low [CO 2 ] ( Fig. 5a–d ). Under normal or increased [CO 2 ], PATROL1-OX plants exhibited similar but slightly higher stomatal conductance compared to the WT. However, this small difference may be sufficient to elevate the CO 2 assimilation rate ( Fig. 5a,b ). We examined the response to desiccation stress in PATROL1-OX plants. The rate of transpirational water loss, evaluated as the fresh weight decrease of the excised PATROL1-OX leaves, resembled that of the WT. This was unlike the response found in the ABA-deficient mutant aba2-1 [35] that showed excessive water loss owing to constitutive stomatal opening ( Fig. 5e ). These results suggested that PATROL1-OX plants control the stomatal aperture efficiently; they could open their stomata wider than the WT to maintain higher CO 2 assimilation rates, and close them to prevent extra water loss depending on the environmental conditions ( Fig. 5 ). 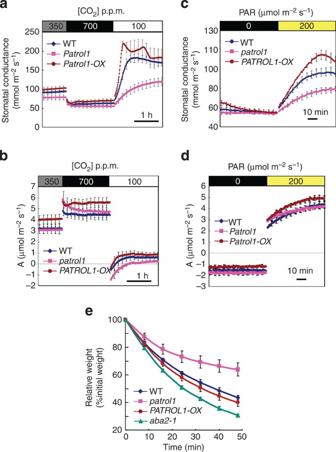Figure 5:PATROL1-overexpressing plants enhance stomatal conductance and CO2assimilation without dessication. (a–d) Stomatal conductance and CO2assimilation rate in response to [CO2] changes (a,b), and to light (c,d). [CO2] and light intensity were changed as indicated. Data represent means±s.e.m. (a,b,n=4;c,d,n=5) from 3–4-week-old plants. (e) Kinetics of water loss from the aerial parts of WT,patrol1,PATROL1-OXandaba2-1plants. Water loss is expressed as the percentage of initial fresh weight. Values are means±s.d. (n=4).patrol1plants show reduced water loss, whilePATROL1-OXplants exhibit normal values. As a wilty mutant control,aba2-1was used. Figure 5: PATROL1 -overexpressing plants enhance stomatal conductance and CO 2 assimilation without dessication. ( a – d ) Stomatal conductance and CO 2 assimilation rate in response to [CO 2 ] changes ( a , b ), and to light ( c , d ). [CO 2 ] and light intensity were changed as indicated. Data represent means±s.e.m. ( a , b , n =4; c , d , n =5) from 3–4-week-old plants. ( e ) Kinetics of water loss from the aerial parts of WT, patrol1 , PATROL1-OX and aba2-1 plants. Water loss is expressed as the percentage of initial fresh weight. Values are means±s.d. (n=4). patrol1 plants show reduced water loss, while PATROL1-OX plants exhibit normal values. As a wilty mutant control, aba2-1 was used. Full size image PATROL1-OX plants exhibit enhanced growth When grown under continuous light for 20 days, patrol1 plants were significantly smaller than the WT ( Fig. 6a,b , analysis of variance (ANOVA), P =1.7 × 10 −11 , post hoc Tukey tests, P =2.4 × 10 −7 ), whereas PATROL1-OX plants were bigger (in terms of above-ground fresh weight; Fig. 6a,b , post hoc Tukey tests, P =0.0496). Thus, plant size correlated with CO 2 assimilation rate under standard [CO 2 ] (350 p.p.m. ; Fig. 5b,d ). Likewise, when grown for 7 weeks under short-day conditions (8 h light, 16 h dark), PATROL1-OX plants were 32% bigger than the WT ( Fig. 6d,e , ANOVA, P =1.17 × 10 −4 , post hoc Tukey tests, P =1.2 × 10 −3 ), although patrol1 rosettes reached the size of WT ones ( Fig. 6d,e , post hoc Tukey tests, P =0.75). Compared to the WT, shorter and longer inflorescence stems were observed in patrol1 and PATROL1-OX , respectively, when grown under continuous light for a month ( Fig. 6c ). Similar results were obtained when plants were grown first under short-day conditions for 7 weeks and then shifted to long-days to induce flowering for 2 more weeks ( Fig. 6f ). Taken together, PATROL1 affects not only stomatal movement but also leaf growth and stem elongation. 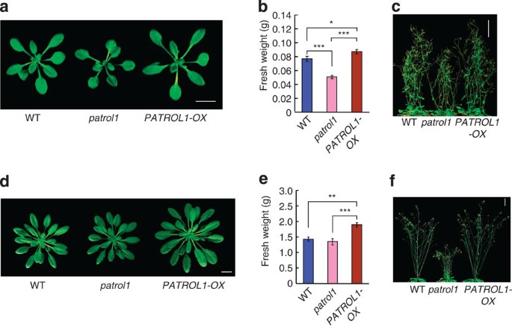Figure 6: Leaf growth is promoted inPATROL1-overexpressing plants. (a–c) Plants grown under continuous light for 20 (a,b), and 34 days (c). (d–f) Plants grown under short-day conditions for 7 weeks (d,e) and further grown under continuous light for 2 weeks (f). (b,e) Fresh weight of aerial parts of the plants. Data are means±s.e.m.;n=21 (b) orn=10 (e). Statistical significance was analysed by ANOVA tests (20 daysP=1.7 × 10−11; 7 weeksP=1.17 × 10−4) followed by apost hocTukey test. Asterisks (*P<0.05, **P<0.005, ***P<0.001) indicate statistical significance. Scale bars=1 cm in (a) and (d), and 5 cm in (c) and (f). Figure 6: Leaf growth is promoted in PATROL1- overexpressing plants. ( a – c ) Plants grown under continuous light for 20 ( a , b ), and 34 days ( c ). ( d – f ) Plants grown under short-day conditions for 7 weeks ( d , e ) and further grown under continuous light for 2 weeks ( f ). ( b , e ) Fresh weight of aerial parts of the plants. Data are means±s.e.m. ; n =21 ( b ) or n =10 ( e ). Statistical significance was analysed by ANOVA tests (20 days P =1.7 × 10 −11 ; 7 weeks P =1.17 × 10 −4 ) followed by a post hoc Tukey test. Asterisks (* P <0.05, ** P <0.005, *** P <0.001) indicate statistical significance. Scale bars=1 cm in ( a ) and ( d ), and 5 cm in ( c ) and ( f ). Full size image In animals, Munc13 proteins are important for synaptic exocytosis and for cytotoxic granule exocytosis in NK cells [36] . Animal Munc13 proteins possess several conserved domains including Ca 2+ -binding sites and/or domains required for homodimerization [36] . Metazoan and fungal MUN domain-containing proteins carry C2 domains suggesting roles in regulating Ca 2+ -dependent exocytosis. In plants, MUN domain-containing proteins are relatively smaller and have no known domains other than MUN [16] . This might suggest that Munc13-like proteins in plants do not need Ca 2+ binding or need other Ca 2+ binding components for its activation. In plants, the functions of Munc13-like genes are generally unknown. In this study, we showed that one of the Arabidopsis Munc13-like genes, PATROL1 , has a role in stomatal responses and growth by regulation of the plasma membrane H + -ATPase. We found that PATROL1 orthologues in higher plants have high identity and similarity to AtPATROL1 including a part adjacent to the MUN domain ( Supplementary Fig. S4 ). These parts may be required for functions unique to plants that need to integrate signals received from the environment including light, CO 2 and humidity. H + -ATPases are known to contribute to stomatal opening, cell elongation, and the growth of root hairs and pollen tubes [5] . Some of the DUF810 family genes have been reported to be expressed in pollen [18] , suggesting functions in pollen germination and tube growth [19] . Thus, these genes may also have a role in H + -ATPase tethering on the plasma membrane in pollen tubes. Endosomes traffic biosynthetic cargo and recycle endocytosed plasma membrane components back to the plasma membrane. We showed that PATROL1 resides in the endosome and moves to and from the plasma membrane in response to environmental stimuli ( Fig. 2 ). Under light and well-watered conditions that induce stomatal opening, PATROL1 mainly was found close to the plasma membrane, whereas under dark or dry conditions that induce stomatal closure, PATROL1 moved away from the plasma membrane ( Fig. 2 ). The AHA1 in the plasma membrane was always associated with PATROL1 on the inside of the plasma membrane ( Fig. 4 ). These facts are consistent with the function of PATROL1 in tethering H + -ATPases to the plasma membrane. Stomatal movements by guard-cell swelling or shrinking require changes of guard-cell surface area through exocytotic addition or endocytotic retrieval of membrane [37] , [38] . When stomata open, intracellular vesicles incorporate with the plasma membrane and PATROL1 may be carried with them to tether H + -ATPases into the plasma membrane. In plasma membrane H + -ATPases, changes in transcriptional levels are often uncoupled from changes in protein activities and/or proton fluxes [6] . It is therefore likely that post-translational modifications determine H + -ATPase activity. Phosphorylation of H + -ATPases and the phosphorylation-dependent binding of 14-3-3 protein are well-studied examples of post-translational regulation [5] . Modifications of the H + -ATPase concentration in the plasma membrane are an alternative means to control total activity, but few studies addressed this alternative regulatory pathway [6] . A nonsense mutation just before the MUN domain of PATROL1 ( Fig. 1d ) resulted in irregular pattern of AHA1 distribution ( Fig. 3a–e ). In addition, patrol1 showed defects in FC-, low CO 2 - and light-induced stomatal opening ( Figs 3f , 5a,c ), which supports the notion that the translocation of H + -ATPases to the plasma membrane is an essential process in stomatal function that is controlled by PATROL1. Furthermore, we showed that higher CO 2 assimilation rates increase biomass production in PATROL1 -overexpressing plants. An Arabidopsis SNARE protein, syntaxin SYP121, functions in the anchoring of K + channels to the plasma membrane through direct physical interaction [39] . The syp121 mutant exhibits delayed stomatal opening and develops similar or smaller rosettes than the WT depending on environmental conditions [30] , similar to patrol1 . This seems to indicate that membrane traffic generally controls stomatal movement, and consequently, plant growth. Dominant-negative Sp2 fragments of SYP121 from Arabidopsis and maize do not affect the plasma membrane delivery of the H + -ATPase PMA2 [40] . Taken together, SNARE proteins select their target plasma membrane proteins directly. PATROL1 may select its target H + -ATPases indirectly by interacting with specific SNARE proteins and control the total amount of the plasma membrane H + -ATPases. In this study, the patrol1 mutation severely impaired the localization of AHA1 but did not affect that of KAT1, indicating that the target SNARE protein PATROL1 associates with may be different from SYP121. Auxin, a plant growth hormone, inhibits endocytosis of plasma membrane proteins and increases the density of H + -ATPases in the PM [41] . H + -ATPase acidifies the apoplast and loosens the cell wall leading to cell expansion [42] . As PATROL1 is expressed in the entire plant ( Supplementary Fig. S4 ), an increased accumulation of H + -ATPases in the plasma membrane of various cell types may contribute to the enhanced growth in PATROL1-OX ( Fig. 6 ). The constitutive activation of H + -ATPases induces stomatal opening, but plants with continuously opened stomata often show comparatively small size and increased susceptibility to drought stress [7] , [43] . PATROL1-OX exhibited normal resistance against water loss ( Fig. 5e ). The ability to prevent water loss may contribute to the increased biomass production in PATROL1-OX . Overexpression of H + -ATPase genes does not always enhance growth because of the downregulation of H + -ATPase activity induced by the overexpression of its gene [43] , [44] . The nature of this feedback mechanism has not been elucidated yet. Similarly, overexpression of AHA1 did not induce biomass increase and rather decreased biomass production in this study ( Supplementary Fig. S7 ). On the contrary, overexpression of PATROL1 increased biomass even in an AHA1 overexpression background ( Supplementary Fig. S7 ). This suggests that PATROL1 is required for efficient biomass production by localizing the proper amount of H + -ATPase to the plasma membrane without downregulating its activity. Stomatal opening in response to environmental signals in PATROL1- overexpressing plants was rapid ( Fig. 5 , Supplementary Fig. S8 ), suggesting that PATROL1 may facilitate H + -ATPase activation. Highly conserved PATROL1 orthologues appear commonly in higher plants ( Fig. 1e , Supplementary Fig. S3 ). Taken together, our findings suggest that increases in biomass production in various plant species of interest may be achievable through manipulations of the function of PATROL1 and related genes. Plant material and growth conditions All Arabidopsis lines used in this study, including a transgenic line expressing SLAC1–GFP [25] , were derived from the Columbia (Col-0) background. EMS-mutagenized Col M 2 seeds were purchased from Lehle Seeds (Round Rock, TX, USA). Plants were grown on solid 1/2 MS medium for 18 days in a growth chamber (constant white light of 80 μmol m –2 s –1 at 22 °C, 60% RH), and then transplanted into vermiculite pots supplemented with mineral nutrients. Under short-day condition, plants were grown on commercial soil (Supermix A, Sakata, Japan) in a growth chamber (8 h light of 127 μmol m –2 s –1 and 16 h dark at 23 °C, 60% RH). Thermal imaging Three-week-old plants were transferred to a growth cabinet (constant white light of 40 μmol m –2 s –1 at 22 °C, 43% RH) equipped with an automatic CO 2 control unit (FR-SP, Koito) [9] . Thermal images of plants were captured under different [CO 2 ] conditions using a thermography apparatus (TVS-8500, Nippon Avionics) [9] . Stomatal aperture response analysis Three-week-old plants were incubated at the indicated [CO 2 ] in a growth cabinet. Abaxial epidermal peels of the plants were taken from the sixth or seventh leaf and were used immediately for aperture determination [9] . In FC treatment, epidermal peels were floated on a test medium containing 10 mM KCl, 10 mM Mes-KOH and 50 μM CaCl 2 (pH 6.15) and were incubated in the growth chamber. FC was added to the solution after 1 h of illumination and stomatal apertures were measured 2 h later [9] . The stomatal aperture was observed in epidermal peels with a digital camera attached to a microscope (BH2, Olympus, Tokyo Japan). Stomatal conductance measurement Gas exchange was measured on the aerial part of the 24-day-old seedlings using gas exchange systems (GFS3000, Heinz Walz, Effeltrich, Germany) equipped with a 3010-A Arabidopsis chamber [45] . The GFS3000 system was connected with a PC with data acquisition software (GFS-Win). The Arabidopsis cuvette was exposed to a light intensity of 200 μmol m –2 s –1 provided by a special artificial light (LED-Array/PAMFluorometer 3055-Fl, Heinz Walz, Effeltrich, Germany), with relative humidity and air temperature set to 50% and 22 °C, respectively. Measurements were made every minute. Transgene construction For functional complementation of the patrol1 mutant, a fragment containing full-length At5g06970 cDNA (accession number AY090450) was prepared from the RAFL 09-69-H21 clone, which was obtaind from RIKEN BioResource Center, Tsukuba, Japan, by digestion with Not I and Bam HI and subcloning into the vector pBluescript II KS + . A Sal I- Bam HI fragment including the cDNA was cloned into the T-DNA vector pPZP2Ha3(−) [46] . For the production of 35S: GFP–PATROL1 , the 35S promoter: GFP fragment with a glycine linker obtained by PCR using primers 5′-GGGCCCCTCGAGCCCCTCAGAAGACCAGAGGGC-3′ and 5′-TACCGGTAGC ACCTCCACCTCC CTTAT-3′ (the glycine linker site is underlined) with pKS(+) GFP – OsGK1 [47] as a template, was inserted into pGEM-T Easy vector (Promega) to produce pG-35S: GFP . A DNA fragment containing the PATROL1 ORF, obtained by PCR using primers 5′-GACCGGTATGGAAGAAGAAAATGCTGTC-3′ and 5′-GAGCTCCCCGGGGATCGTAAACTACAAACATTTGTA-3′, was inserted into the pGEM-T Easy vector to produce pG- PATROL1 . The Sac II– Age I fragment of pG-35S:GFP1 containing the CaMV 35S promoter and GFP cDNA was inserted into the Sac II/ Age I sites of pG- PATROL1 to produce pG-35S: GFP–PATROL1 . The Xho I- Sma I fragment of pG-35S: GFP–PATROL1 was inserted into the Xho I/ Sma I sites of pPZP2H-lac. For 35S: GFP–AHA1 , a DNA fragment containing AHA1 ORF was obtained by PCR using primers 5′-TATAAGGGAGGTGGAGGTGCTATGTCAGGTCTCGAAG-3′ and 5′-AGAACTAGTGGATCCCCCGGGTTTTAGAATTAAATTTAAATATTAT-3′. The Age I/ Sma I fragment obtained by digestion of the PCR-amplified AHA1 was inserted together with an Xho I/ Age I fragment of 35S:GFP into the Xho I/ Sma I sites of pPZP2H-lac [46] . For 35S:RFP–AHA1 production, RFP was obtained by PCR using primers 5′-AGGATCCATGGCCTCCTCCGAGGA-3′ and 5′-CATAGCACCTCCACCTCCCTTATA GGCGCCGGTGGAGTGGCGGC-3′ with mRFP plasmid as a template. A DNA fragment containing AHA1 ORF was obtained by PCR using primers 5′-GCCGCCACTCCACCGGCGCCTATAAGGGAGGTGGAGGTGCT-3′ and 5′-AGAACTAGTGGATCCCCCGGGTTTTAGAATTAAATTTAAATATTAT-3′. A DNA fragment containing RFP–AHA1 was obtained by PCR using primers 5′-AGGATCCATGGCCTCCTCCGAGGA-3′ and 5′-AGAACTAGTGGATCCCCCGGGTTTTAGAATTAAATTTAAATATTAT-3′ with RFP and AHA1 fragments as templates. The Bam HI/ Sma I fragment obtained by digestion of the PCR-amplified RFP–AHA1 was inserted into Bam HI/ Sma I sites of pPZP2Ha3. A pPATROL1::GUS construct was obtained by amplifying 2 kb of the PATROL1 promoter region from genomic DNA using the oligonucleotides 5′-CGGTCGACACAACCACTAGC-3′ and 5′-GGATCCCTCGATCCAGCTGCAATAAT-3′; the product was then inserted into the pGEM-T Easy Vector. A Sal I- Bam HI fragment including the PATROL1 promoter sequences was cloned into the Sal I and Bam HI sites of pBI101. Immunohistochemical analysis Immunohistochemical detection of the plasma membrane H + -ATPase in the epidermis was performed as described [33] with minor modifications. Plants were incubated under low CO 2 (<100 p.p.m.) for at least an hour. The abaxial epidermis of the rosette leaves was peeled with a forceps, and immediately incubated in 4% ( w / v ) formaldehyde in fixation buffer for 2.5 h at room temperature. The fixed epidermis was rinsed with water and attached to an MAS-coated glass slide. The samples were digested by cellulase solutions (1% Cellulase Onozuka R-10 (Yakult) and 0.1% Macerozyme R-10 (Yakult) in PBS) for 20 min at 37 °C. The samples were rinsed twice with PBS and permeabilized with 0.5% ( w / v ) Triton X-100 for 30 min, and then were blocked with 3% bovine serum albumin Fraction V. The samples were incubated with anti-plasma membrane H + -ATPase (anti-AHA; Cosmo Bio) at a dilution of 1:1,000 for 16 h. The secondary antibody used here was Alexa Fluor 594 goat anti-rabbit IgG (Invitrogen; 1:500) for 3 h in the dark. After washing the samples, each specimen was mounted on a glass slide with 50% (v/v) glycerol. Microscopy The leaves were covered by a glass slide and observed under a fluorescence microscope (IX70, Olympus) equipped with an UPlanApo × 100/1.35 oil iris objective lens and a confocal scanning head (CSU10, Yokogawa). For staining endosomes, the seedlings were treated with 33 μM FM4-64 (Invitrogen), for 2 min and then washed with basal buffer (5 mM MES-Tris, 10 mM CaCl 2 , 50 mM KCl, pH6.5). The hypocotyl epidermis was examined immediately. GFP and FM4-64 were excited with a laser (HPU-50101-PFS2; Furukawa) at 488 nm and the fluorescence was detected with a cooled CCD camera head system (CoolSNAP HQ, Photometrics) through a 524–546 nm band-pass filter (FF01-535/22-25, Semrock) for GFP, and a 604–644 band-pass filter (FF01-624/40-25, Semrock) for FM4-64. For light treatment, the leaves were irradiated with 200 μmol m −2 s −1 white light for 30 min with a cold light illumination system (LG-PS2, Olympus). In order to prevent drying, 3-mm-thick 1% agarose gels with basal buffer were placed onto the leaves [48] . For osmotic treatments, leaves were incubated in basal buffer (120 mOsM) or basal buffer with 0.4 M Mannitol (530 mOsM) for 15–30 min. Fluorescence from the secondary antibody, Alexa Fluor 594, was collected using a 561 nm laser (85-YCA-025-040, CVI Melles Griot) for excitation and a 580–600 nm band-pass filter (FF01-590/20-25, Semrock) for emission. For quantification of the Alexa Fluor 594 intensity, we measured the background-subtracted mean intensity in the signal regions that were segmented with Otsu’s thresholding algorithm [49] . Isolation of guard cell and mesophyll cell protoplasts GCPs from 600 to 1,200 leaves were isolated as described [25] . MCPs were isolated as described elsewhere [50] with some modifications. Twenty leaves from a 3–4-week-old plant were cut into 1-mm strips using a razor blade. Leaf strips were transferred into enzyme solution (5 mM MES (pH 5.6) containing 1% ( w / v ) cellulase R-10, 0.4% ( w / v ) macerozyme R-10, 0.1% ( w / v ) polyvinylpyrrolidone K-30 (PVP-40), 0.6 M mannitol, 0.5 mM CaCl 2 , 0.5 mM MgCl 2 and 0.2% ( w / v ) BSA), and incubated at 24 °C for 2 h. Protoplasts were filtered through double layers of 50 μm nylon mesh and collected by centrifugation at 140 g for 4 min. GCP and MCP protoplasts were subjected to density gradient centrifugation at 200 g for 20 min using Histopaque-1077. The purity of the GCPs and MCPs were always higher than 97 and 99%, respectively. Transgene expression analysis Histochemical staining of GUS activity in pPATROL1::GUS transformants was assayed with 5-bromo-4-chloro-3-indolyl-D-glucuronide as a substrate [9] . To obtain tissue sections, GUS-stained samples were embedded in Technovit 8100 according to the manufacturers’ instructions (Heraeus Kulzer GmbH, Wehrheim, Germany). A rotary microtome (Yamato Kohki) was used to cut 10-μm-thick sections. Total RNA from plant tissues or protoplasts were extracted and single-stranded cDNA synthesized from total RNA was used as RT-PCR templates according to the method described by Sugimoto et al. [51] . The RT-PCR primers for PATROL1 were 5′-CTTCAGAGATATCGCCGGGA-3′ and 5′-CAATCCTGATGAGCTCTGAG-3′. An amplified 700-bp fragment of the EF1α cDNA was used as an internal standard [9] . Expression of PATROL1 in guard cell and mesophyll cell protoplasts was examined by RT-PCR. The HT1 gene was used as a guard-cell-specific expression control [9] , and the CBP marker gene was used as a mesophyll-cell-specific expression control [52] using primers 5′-CTTATCTGGAGGTGCCACAA-3′ and 5′-CCTCACTCTTTCTTGGATAAC-3′. Water-loss measurement The weight of detached rosette leaves was determined every 8 min. Three-week-old 1/2 MS plate-grown plants were used. Water loss was expressed as the percentage of initial fresh weight. How to cite this article: Hashimoto-Sugimoto, M. et al. A Munc13-like protein in Arabidopsis mediates H + -ATPase translocation that is essential for stomatal responses. Nat. Commun. 4:2215 doi: 10.1038/ncomms3215 (2013).